E2F1-dependent miR-421 regulates mitochondrial fragmentation and myocardial infarction by targeting Pink1 Mitochondrial fragmentation plays an important role in the progression of cardiac diseases, such as myocardial infarction and heart failure. Mitochondrial network is controlled by many factors in different cell types. Here we show that the interplay between E2F1, miR-421 and Pink1 regulates mitochondrial morphology and cardiomyocyte cell death. Pink1 reduces mitochondrial fragmentation and protects cardiomyocyte from apoptosis. On the other hand, miR-421 promotes cardiomyocyte mitochondrial fragmentation, apoptosis and myocardial infarction by suppressing Pink1 translation. Finally, we show that transcription factor E2F1 activates miR-421 expression. Knocking down E2F1 suppresses mitochondrial fragmentation, apoptosis and myocardial infarction by affecting miR-421 levels. Collectively, these data identify the E2F1/miR-421/Pink axis as a regulator of mitochondrial fragmentation and cardiomyocyte apoptosis, and suggest potential therapeutic targets in treatment of cardiac diseases. Cardiovascular diseases remain the leading cause of morbidity and mortality worldwide [1] . Heart failure is the common end stage of cardiovascular diseases and represents a decline in cardiac function. Heart failure involves the impairment of cardiomyocytes in energy metabolism, calcium homeostasis, reactive oxygen species production and cell death [2] , [3] , [4] . Since mitochondria are the major ATP and reactive oxygen species production organelle in cardiomyocytes, mitochondrial malfunction is tightly related to cardiovascular diseases and contributes to heart failure. Mitochondria function and morphology are tightly associated with each other. Mitochondria constantly undergo fission and fusion. Fission leads to the formation of small round mitochondria and promotes cell apoptosis, whereas fusion results in mitochondria elongation and plays a protective role in cardiomyocytes maintenance [5] . Although emerging evidences demonstrate that mitochondrial fission and fusion machinery are important for maintaining cardiac function [6] , [7] , [8] , little work suggests the transcriptional control of mitochondrial network regulators. And unveiling the mechanism of mitochondrial network regulation will provide a novel therapeutic strategy for heart failure. Pink1 is a mitochondrial targeted Ser/Thr kinase, mutation of which is associated with parkinsonism [9] . Under the condition of mitochondrial depolarization, the mitochondrial import is damaged and Pink1 accumulates on the mitochondrial surface. Pink1 recruits and intermediates Parkin phosphorylation, which results in the Parkin translocation from the cytosol to mitochondria [10] , [11] . The Pink1/Parkin pathway is tightly associated with the mitochondrial fission and fusion machinery. The dysfunction of this signalling usually leads to neurodegeneration. Pink1 loss of function increases mitochondrial fission in Drosophila and mammalian neurons [12] . Recent study has also shown that overexpression of Pink1 in HL-1 cardiac cells reduces cell death post ischaemia/reperfusion (I/R), and Pink1-knockout (KO) mice are more susceptible to I/R injury compared with wild-type (WT) mice [13] . Although the role of Pink1 on mitochondrial morphology has been studied in Drosophila , and the repressive role of Pink1 on myocardial cell death has also been reported, it is yet unclear whether pink1 is able to regulate mitochondrial fragmentation in cardiomyocytes. MicroRNAs (miRNAs) are a class of short single-stranded non-coding endogenous RNAs and act as negative regulators of gene expression by inhibiting messenger RNA (mRNA) translation or promoting mRNA degradation [14] , [15] . Approximately, about one-third of functional genes are regulated by miRNA [16] . MiRNAs participate in a variety of biological process, such as proliferation, differentiation, metabolism and cell death. More and more studies demonstrate a key role of miRNA dysregulation in cardiovascular disease process and their involvement in heart failure [17] , [18] . However, whether miRNAs maintain cardiac function by regulating mitochondria dynamics remains speculated. Excavating the function of miRNA in the mitochondria might shed new light on the machinery that underlies mitochondrial regulation and promote the effective therapy of cardiovascular diseases. E2F1 is pivotal for cardiac function and mainly affect the metabolism of cardiomyocytes. E2F1 KO mice have lower blood glucose levels and enhanced glucose oxidation, and show a variety of age-related defects [16] . Mutation of E2F1 can induce congestive heart failure [19] . I/R injury causes an increase in E2F1 protein levels, and the deletion of E2F1 reduces infarct size during I/R injury [20] . These studies further substantiate the notion that E2F1 plays an important role in the pathological development of heart disease. However, it is not yet clear whether E2F1 participates in the regulation of mitochondrial dynamics in cardiomyocytes. Our present study confirms and extends previous findings that Pink1 is involved in the regulation of the mitochondrial network in cardiomyocytes [13] . Pink1 inhibits mitochondrial fragmentation and apoptosis in cardiomyocytes. And Pink1-transgenic mice exhibit reduced myocardial infarction sizes on I/R injury in vivo . In searching for the mechanism by which Pink1 is downregulated under pathologic condition, we identify that miR-421 participates in the suppressing of Pink1 translation. MiR-421 initiates mitochondrial fragmentation, apoptosis and myocardial infarction by downregulating Pink1. We further find that E2F1 can transcriptionally activate miR-421 expression and, thus, regulate mitochondrial fragmentation and apoptosis. Our results reveal a novel mitochondrial regulating model that is composed of E2F1, miR-421 and Pink1. Modulation of their levels may represent a novel approach for interventional treatment of myocardial infarction and heart failure. Pink1 inhibits mitochondrial fragmentation and apoptosis To test whether Pink1 participates in the regulation of mitochondrial fragmentation and apoptosis in cardiomyocytes, we treated cardiomyocytes with H 2 O 2 to induce mitochondrial fragmentation and apoptosis. The expression levels of Pink1 were downregulated in response to H 2 O 2 treatment ( Fig. 1a ). We then tested whether Pink1 was involved in the occurrence of mitochondrial fragmentation. Enforced expression of Pink1 efficiently attenuated the decrease of Pink1 induced by H 2 O 2 treatment ( Fig. 1b ). Enforced expression of Pink1 also attenuated mitochondrial fragmentation induced by H 2 O 2 as revealed by the analysis of mitochondrial morphology and the counting of the cells with fragmentation ( Fig. 1c ; Supplementary Fig.1 ). Furthermore, Pink1 also attenuated H 2 O 2 -induced apoptosis analysed by TdT-mediated dUTP nick end labelling assay ( Fig. 1c ). Taken together, these results suggest that Pink1 participates in the regulation of mitochondrial fragmentation and apoptosis in cardiomyocytes. 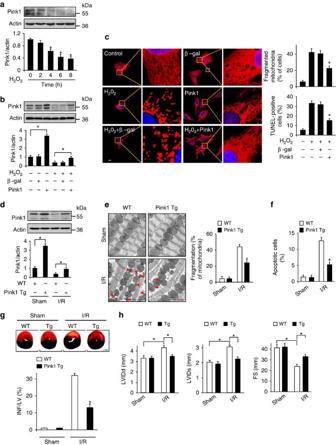Figure 1: Pink1 inhibits mitochondrial fragmentation and apoptosis. (a) Cardiomyocytes were treated with 150 μM H2O2at indicated time. Pink1 levels were analysed by immunoblot. Data are shown as mean±s.e.m. of three independent experiments. *P<0.05 versus untreated group in Student’st-test. (b) Cardiomyocytes were infected with adenoviral Pink1 and β-gal, then exposed to H2O2. Pink1 levels were analysed by immunoblot. Data are shown as mean±s.e.m. of three independent experiments. Analysis was performed with one-way analysis of variance (ANOVA) followed by Tukey–Kramerpost hocanalysis. *P<0.05. (c) Cardiomyocytes were treated as described inb. The cells with fragmented mitochondria were counted (right panel, upper panel). Bar=20 μm. TdT-mediated dUTP nick end labelling (TUNEL) was employed to analyse apoptotic cells (right panel, lower panel). Data are shown as mean±s.e.m. of three independent experiments. Analysis was performed with one-way ANOVA followed by Tukey–Kramerpost hocanalysis. *P<0.05 versus H2O2alone. (d) WT and Pink1-transgenic mice were subjected to I/R as described in Methods. Pink1 levels were detected by immunoblot. Data are shown as mean±s.e.m. of four independent experiments. Analysis was performed with one-way ANOVA followed by Tukey–Kramerpost hocanalysis. *P<0.05. (e,f) Pink1-transgenic mice represent attenuated mitochondrial fragmentation and apoptosis on I/R injury. The fragmented mitochondria were shown ine. TUNEL assay was performed to detect apoptotic cells (f). Data are shown as mean±s.e.m. of six independent experiments. Analysis was performed with one-way ANOVA followed by Tukey–Kramerpost hocanalysis. *P<0.05 versus WT+I/R. (g) Pink1-transgenic mice show attenuated myocardial infarct sizes in response to I/R. The upper panels are representative photos of midventricular myocardial slices. The lower panel shows infarct sizes. LV, left ventricle; INF, infarct area. Data are shown as mean±s.e.m. of six independent experiments. Analysis was performed with one-way ANOVA followed by Tukey–Kramerpost hocanalysis. *P<0.05 versus WT+I/R. Bar=2mm. (h) Pink1-transgenic mice present markedly preserved cardiac function after I/R. Transthoracic echocardiographic analysis was performed. Data are shown as mean±s.e.m. of six independent experiments. Analysis was performed with one-way ANOVA followed by Tukey–Kramerpost hocanalysis. *P<0.05. Figure 1: Pink1 inhibits mitochondrial fragmentation and apoptosis. ( a ) Cardiomyocytes were treated with 150 μM H 2 O 2 at indicated time. Pink1 levels were analysed by immunoblot. Data are shown as mean±s.e.m. of three independent experiments. * P <0.05 versus untreated group in Student’s t -test. ( b ) Cardiomyocytes were infected with adenoviral Pink1 and β-gal, then exposed to H 2 O 2 . Pink1 levels were analysed by immunoblot. Data are shown as mean±s.e.m. of three independent experiments. Analysis was performed with one-way analysis of variance (ANOVA) followed by Tukey–Kramer post hoc analysis. * P <0.05. ( c ) Cardiomyocytes were treated as described in b . The cells with fragmented mitochondria were counted (right panel, upper panel). Bar=20 μm. TdT-mediated dUTP nick end labelling (TUNEL) was employed to analyse apoptotic cells (right panel, lower panel). Data are shown as mean±s.e.m. of three independent experiments. Analysis was performed with one-way ANOVA followed by Tukey–Kramer post hoc analysis. * P <0.05 versus H 2 O 2 alone. ( d ) WT and Pink1-transgenic mice were subjected to I/R as described in Methods. Pink1 levels were detected by immunoblot. Data are shown as mean±s.e.m. of four independent experiments. Analysis was performed with one-way ANOVA followed by Tukey–Kramer post hoc analysis. * P <0.05. ( e , f ) Pink1-transgenic mice represent attenuated mitochondrial fragmentation and apoptosis on I/R injury. The fragmented mitochondria were shown in e . TUNEL assay was performed to detect apoptotic cells ( f ). Data are shown as mean±s.e.m. of six independent experiments. Analysis was performed with one-way ANOVA followed by Tukey–Kramer post hoc analysis. * P <0.05 versus WT+I/R. ( g ) Pink1-transgenic mice show attenuated myocardial infarct sizes in response to I/R. The upper panels are representative photos of midventricular myocardial slices. The lower panel shows infarct sizes. LV, left ventricle; INF, infarct area. Data are shown as mean±s.e.m. of six independent experiments. Analysis was performed with one-way ANOVA followed by Tukey–Kramer post hoc analysis. * P <0.05 versus WT+I/R. Bar=2mm. ( h ) Pink1-transgenic mice present markedly preserved cardiac function after I/R. Transthoracic echocardiographic analysis was performed. Data are shown as mean±s.e.m. of six independent experiments. Analysis was performed with one-way ANOVA followed by Tukey–Kramer post hoc analysis. * P <0.05. Full size image To understand the pathophysiological role of Pink1, we detected whether Pink1 was involved in the pathogenesis of myocardial infarction in the animal model. We generated transgenic mice with cardiac-specific overexpressed Pink1 ( Supplementary Fig. 2a–c ). These mice developed normally to adulthood without significant alterations in terms of phenotype and cardiac function under physiological condition. Pink1-transgenic mice exhibited elevated Pink1 levels, compared with the WT group on I/R injury ( Fig. 1d ). Furthermore, Pink1-transgenic mice showed a reduction in mitochondrial fragmentation ( Fig. 1e ) and apoptosis ( Fig. 1f ) in response to I/R injury. Myocardial infarction size in Pink1-transgenic mice also decreased remarkably, compared with the WT group on I/R injury ( Fig. 1g ). The cardiac function and mitochondrial function were ameliorated in the Pink1-transgenic mice group ( Fig. 1h ; Supplementary Fig. 2d ). In addition, we also demonstrated that the mitochondrial fusion was increased in cardiomyocytes from the transgenic mice ( Supplementary Fig. 2e ). Thus, it appears that Pink1 is able to inhibit mitochondrial fragmentation, apoptosis and myocardial infarction in the heart. Next, we explored how Pink1 altered mitochondrial morphology in our model. Previous reports showed that Parkin requires Pink1 for mitochondrial translocation and recruitment [21] , [22] . Thus, we tested whether Parkin was also recruited to the mitochondria or it was a separate pathway in our signalling axis. We detected Parkin expression in mitochondria in response to H 2 O 2 or I/R treatment. And our results showed that there was no difference of expression between the control group and treatment group ( Supplementary Fig. 3a ; Supplementary Fig. 3b ), suggesting that Parkin was in a separate pathway in our model. Previous reports have indicated that Pink1 kinase activity is tightly related to mitochondrial function. It has been reported that Pink1 phosphorylates Miro and participates in mitochondrial depolarization [23] . Pink1 phosphorylates Mfn2 and mediates mitochondrial degradation [24] . Pink1 binds and colocalizes with TRAP1 in the mitochondria. Also, Pink1 phosphorylates TRAP1 both in vitro and in vivo [25] . Thus, we tested whether Pink1 kinase activity is also required for mitochondrial fragmentation and apoptosis pathway in cardiomyocytes. And our results showed that kinase dead Pink1 mutation lost the ability to protect against H 2 O 2 -induced mitochondrial fragmentation ( Supplementary Fig. 3c ) and apoptosis ( Supplementary Fig. 3d ), indicating that the protective effects of Pink1 on mitochondrial fragmentation and apoptosis depend on its kinase activity. Then, we further tested whether Miro, Mfn2 or TARP1 could be downstream targets in our signal pathway. We detected the phosphorylation levels of Miro, Mfn2 and TRAP1. We found that there was no significant change in the phosphorylation levels of Miro and Mfn2 ( Supplementary Fig. 4a,b ) and only the phosphorylation level of TRAP1 was decreased ( Supplementary Fig. 4c ). These results indicated that TRAP1, but not Miro or Mfn2, might participate in our Pink1-dependent cardiomyocytes mitochondrial fragmentation and apoptosis pathway. To provide further evidence supporting the role of Pink1 in regulation of TRAP1 phosphorylation, we examined the effect of short interfering RNA (siRNA)-mediated Pink1 knockdown on TRAP1 phosphorylation. As shown in Supplementary Fig. 4d , phosphorylation of endogenous TRAP1 was significantly decreased in cardiomyocytes transfected with Pink1 siRNA. We next examined the effects of WT or mutant Pink1 on the in vivo phosphorylation of endogenous TRAP1 in response to H 2 O 2 treatment. As shown in Supplementary Fig. 4e , overexpression of WT Pink1 inhibited the decrease of TRAP1 phosphorylation in response to H 2 O 2 treatment, and the ability of Pink1 to promote in vivo TRAP1 phosphorylation was abolished by the kinase dead Pink1 mutant. To further test whether TRAP1 is a downstream target of Pink1 that participated in Pink1-dependent mitochondrial fragmentation signal pathway, we investigated the effect of siRNA-mediated TRAP1 knockdown on the protective function of Pink1. TRAP1-targeting siRNA was used to reduce the expression of endogenous TRAP1 in cardiomyocytes ( Supplementary Fig. 4f ). Analysis of mitochondrial fragmentation and apoptosis revealed that knockdown of TRAP1 inhibited the protective effects of Pink1 on H 2 O 2 -induced mitochondrial fragmentation ( Supplementary Fig. 4g ) and apoptosis ( Supplementary Fig. 4h ). Taken together, these results provide evidence supporting a role of TRAP1 as the downstream effector of Pink1 in protection against H 2 O 2 -induced mitochondrial fragmentation and apoptosis. In the future, we intend to carry out more rigorous studies on the identification of potential targets of Pink1 and clarify the most promising molecular effectors to be investigated for cardiovascular diseases. miR-421 participates in the regulation of Pink1 expression MiRNAs are a class of small non-coding RNAs and act as negative regulators of gene expression. To explore the underlying mechanism by which Pink1 is downregulated on H 2 O 2 and I/R injury, we tested whether Pink1 can be regulated by miRNA. We first screened some miRNAs by quantitative real time PCR (qRT–PCR) analysis, function of which had been reported in the past few years. Among several miRNAs, miR-421 levels were significantly upregulated on H 2 O 2 ( Fig. 2a ; Supplementary Fig. 5a ) and other miRNAs remain unchanged ( Supplementary Fig. 5a ). MiR-421 was also significantly increased in the heart of diseased murine ( Supplementary Fig. 5b ) and human heart failure samples ( Supplementary Fig. 5c ). We compared the expression level of miR-421 and cardiac abundant miR-1, and found that the expression level of miR-421 was less than one-third of the miR-1 expression in the mouse heart ( Supplementary Fig. 5d ). 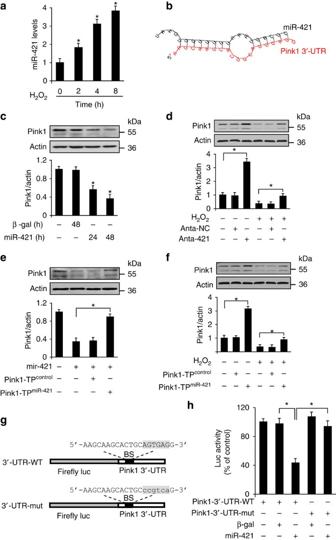Figure 2: miR-421 participates in the regulation of Pink1 expression. (a) MiR-421 levels were analysed by qRT–PCR. Data are shown as mean±s.e.m. of four independent experiments. *P<0.05 versus untreated group in Student’st-test. (b) Putative miR-421-binding site in the 3′-UTR region of Pink1. (c) Cardiomyocytes were infected with adenoviral miR-421 or β-gal. The levels of Pink1 were analysed by immunoblot. Data are shown as mean±s.e.m. of three independent experiments. *P<0.05 versus untreated group in Student’st-test. (d) Cardiomyocytes were transfected with miR-421 antagomir (anta-421) or the antagomir negative control (anta-NC), then exposed to H2O2. The levels of Pink1 were analysed by immunoblot. Data are shown as mean±s.e.m. of three independent experiments. Analysis was performed with one-way analysis of variance (ANOVA) followed by Tukey–Kramerpost hocanalysis. *P<0.05. (e) Pink1 target protector attenuates the reduction of Pink1 induced by miR-421. Cardiomyocytes were infected with adenoviral miR-421, then transfected with the target protector (Pink1-TPmiR-421) or the control (Pink1-TPcontrol). Pink1 levels were detected by immunoblot. Data are shown as mean±s.e.m. of three independent experiments. Analysis was performed with one-way ANOVA followed by Tukey–Kramerpost hocanalysis. *P<0.05. (f) Pink1 target protector inhibits H2O2-induced Pink1 downregulation. Cardiomyocytes were transfected with the Pink1-TPmiR-421or Pink1-TPcontrol, and then exposed to H2O2. The levels of Pink1 were analysed by immunoblot. Data are shown as mean±s.e.m. of three independent experiments. Analysis was performed with one-way ANOVA followed by Tukey–Kramerpost hocanalysis. *P<0.05. (g) Pink1 wild-type (WT) 3′-UTR and a mutated 3′-UTR in the miR-421-binding site are shown. (h) miR-421 suppresses Pink1 translation. HEK293 cells were infected with adenoviral miR-421 or β-gal, then transfected with the luciferase constructs of the WT Pink1-3′-UTR (Pink1-3′-UTR-WT) or a mutated Pink1-3′-UTR (Pink1-3′-UTR-mut). The luciferase activity was analysed. Data are shown as mean±s.e.m. of four independent experiments. Analysis was performed with one-way ANOVA followed by Tukey–Kramerpost hocanalysis. *P<0.05. Figure 2: miR-421 participates in the regulation of Pink1 expression. ( a ) MiR-421 levels were analysed by qRT–PCR. Data are shown as mean±s.e.m. of four independent experiments. * P <0.05 versus untreated group in Student’s t -test. ( b ) Putative miR-421-binding site in the 3′-UTR region of Pink1. ( c ) Cardiomyocytes were infected with adenoviral miR-421 or β-gal. The levels of Pink1 were analysed by immunoblot. Data are shown as mean±s.e.m. of three independent experiments. * P <0.05 versus untreated group in Student’s t -test. ( d ) Cardiomyocytes were transfected with miR-421 antagomir (anta-421) or the antagomir negative control (anta-NC), then exposed to H 2 O 2 . The levels of Pink1 were analysed by immunoblot. Data are shown as mean±s.e.m. of three independent experiments. Analysis was performed with one-way analysis of variance (ANOVA) followed by Tukey–Kramer post hoc analysis. * P <0.05. ( e ) Pink1 target protector attenuates the reduction of Pink1 induced by miR-421. Cardiomyocytes were infected with adenoviral miR-421, then transfected with the target protector (Pink1-TP miR-421 ) or the control (Pink1-TP control ). Pink1 levels were detected by immunoblot. Data are shown as mean±s.e.m. of three independent experiments. Analysis was performed with one-way ANOVA followed by Tukey–Kramer post hoc analysis. * P <0.05. ( f ) Pink1 target protector inhibits H 2 O 2 -induced Pink1 downregulation. Cardiomyocytes were transfected with the Pink1-TP miR-421 or Pink1-TP control , and then exposed to H 2 O 2 . The levels of Pink1 were analysed by immunoblot. Data are shown as mean±s.e.m. of three independent experiments. Analysis was performed with one-way ANOVA followed by Tukey–Kramer post hoc analysis. * P <0.05. ( g ) Pink1 wild-type (WT) 3′-UTR and a mutated 3′-UTR in the miR-421-binding site are shown. ( h ) miR-421 suppresses Pink1 translation. HEK293 cells were infected with adenoviral miR-421 or β-gal, then transfected with the luciferase constructs of the WT Pink1-3′-UTR (Pink1-3′-UTR-WT) or a mutated Pink1-3′-UTR (Pink1-3′-UTR-mut). The luciferase activity was analysed. Data are shown as mean±s.e.m. of four independent experiments. Analysis was performed with one-way ANOVA followed by Tukey–Kramer post hoc analysis. * P <0.05. Full size image Further, we analysed the 3′-untranslated region (UTR) of Pink1 using the RNAhybrid program and observed that Pink1 was a potential target of miR-421 ( Fig. 2b ). And Pink1 was conserved across species in the binding site of miR-421 ( Supplementary Fig. 5e ), which promoted us to focus on the function of miR-421. We first tested whether overexpression or knockdown of miR-421 could alter the expression of endogenous Pink1. Our results showed that enforced expression of miR-421 resulted in a reduction of endogenous Pink1 ( Fig. 2c ). In contrast, knockdown of endogenous miR-421 by antagomir induced an increase in Pink1 expression on H 2 O 2 treatment ( Fig. 2d ). To understand whether the effect of miR-421 on Pink1 was specific, we then employed the Target Protector technology [26] . The inhibitory effect of miR-421 on Pink1 expression was reduced in the presence of the target protector ( Fig. 2e ). Pink1 downregulation was attenuated by the target protector in response to H 2 O 2 ( Fig. 2f ). These results indicated that miR-421 can specifically regulate Pink1. We employed the luciferase assay system to test whether miR-421 can influence the translation of Pink1. As shown in Fig. 2h , the luciferase reporter assay revealed that the WT 3′-UTR of Pink1 exhibited a low translation level in the presence of miR-421, whereas the mutated 3′-UTR ( Fig. 2g ) did not show a significant response to miR-421. Taken together, these data suggest that Pink1 is a specific target of miR-421. Our previous report showed that calcineurin-Drp1 axis influenced I/R response [26] , thus we tested whether Drp1 could also act as a target of miR-421. Our results showed that miR-421 had no effect on Drp1 expression and translation activity ( Supplementary Fig. 6a,b ), suggesting that miR-421-regulated mitochondrial fragmentation was not dependent on Drp1. It is well known that numerous pathways function in the I/R response, such as transforming growth factor-β, Wnt and PI3K/Akt [27] , [28] , [29] . Thus, different miRNAs also involved in different signal pathways in I/R response. For example, miR-320 targets to HSP20 in the regulation of cardiac I/R injury [30] . And miR-21 regulates fibroblast metalloprotease-2 in murine myocardial infarction [31] . Also, miR-494 targets to PTEN, ROCK1 and CaMKIIδ in the cardiac I/R injury [32] . In the future, we will unveil more regulators that function in I/R response and provide more valuable therapeutic targets for effective treatment of cardiac diseases. miR-421 regulates mitochondrial fragmentation and apoptosis We explored the functional role of miR-421 in mitochondrial fragmentation and apoptosis. Knockdown of miR-421 by antagomir efficiently attenuated miR-421 levels in response to H 2 O 2 treatment ( Fig. 3a ). Knockdown of miR-421 also attenuated H 2 O 2 -induced mitochondrial fragmentation ( Fig. 3b ) and apoptosis ( Fig. 3c ). These data indicate that knockdown of miR-421 can inhibit mitochondrial fragmentation and apoptosis in cardiomyocytes. 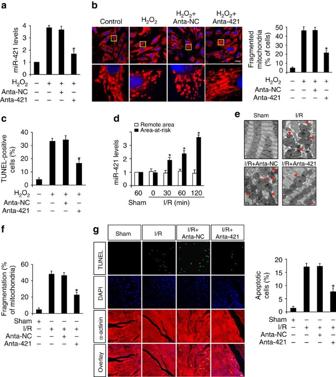Figure 3: miR-421 regulates mitochondrial fragmentation and apoptosis. (a) miR-421 antagomir inhibits the elevation of miR-421 levels on H2O2. Cardiomyocytes were transfected with anta-421 or anta-NC, then exposed to H2O2. Cells were harvested for qRT–PCR analysis of miR-421 levels. Data are shown as mean±s.e.m. of four independent experiments. Analysis was performed with one-way analysis of variance (ANOVA) followed by Tukey–Kramerpost hocanalysis. *P<0.05 versus H2O2alone. (b,c) Knockdown of miR-421 prevents mitochondrial fragmentation and apoptosis induced by H2O2. Cardiomyocytes were treated as described ina, the cells were stained with MitoTracker Red (b), Bar=20 μm. The cells with fragmented mitochondria were counted (b). Apoptosis was analysed by TdT-mediated dUTP nick end labelling (TUNEL) assay (c). Data are shown as mean±s.e.m. of three independent experiments. Analysis was performed with one-way ANOVA followed by Tukey–Kramerpost hocanalysis. *P<0.05 versus H2O2alone. (d) miR-421 is upregulated in response to I/R injury. Mice were subjected to I/R as described in Methods. MiR-421 levels were detected by qRT–PCR. Data are shown as mean±s.e.m. of five independent experiments. *P<0.05 versus sham in Student’st-test. (e,f) Knockdown of miR-421 attenuates mitochondrial fragmentation on I/R. Adult male C57BL/6 mice (8 weeks old) were delivered in 3 consecutive days, intravenous injections of miR-421 antagomir (anta-421) or antagomir control (anta-NC) at doses of 30 mg kg−1body weight. Three days after injection, the mice were subjected to I/R. The fragmented mitochondria were shown ineand counting of the fragmented mitochondria was shown inf. Data are shown as mean±s.e.m. of six independent experiments. Analysis was performed with one-way ANOVA followed by Tukey–Kramerpost hocanalysis. *P<0.05 versus I/R alone. (g) Knockdown of miR-421 attenuates apoptosis on I/R. Counting of the apoptotic cell was shown. TUNEL-positive cardiomyocyte nuclei (apoptotic cells) were green. Nuclei stained by DAPI showed blue. Cardiomyocytes were labelled with α-actinin. Data are shown as mean±s.e.m. of six independent experiments. Analysis was performed with one-way ANOVA followed by Tukey–Kramerpost hocanalysis. *P<0.05 versus I/R alone. DAPI, 4,6-diamidino-2-phenylindole. Figure 3: miR-421 regulates mitochondrial fragmentation and apoptosis. ( a ) miR-421 antagomir inhibits the elevation of miR-421 levels on H 2 O 2 . Cardiomyocytes were transfected with anta-421 or anta-NC, then exposed to H 2 O 2 . Cells were harvested for qRT–PCR analysis of miR-421 levels. Data are shown as mean±s.e.m. of four independent experiments. Analysis was performed with one-way analysis of variance (ANOVA) followed by Tukey–Kramer post hoc analysis. * P <0.05 versus H 2 O 2 alone. ( b , c ) Knockdown of miR-421 prevents mitochondrial fragmentation and apoptosis induced by H 2 O 2 . Cardiomyocytes were treated as described in a , the cells were stained with MitoTracker Red ( b ), Bar=20 μm. The cells with fragmented mitochondria were counted ( b ). Apoptosis was analysed by TdT-mediated dUTP nick end labelling (TUNEL) assay ( c ). Data are shown as mean±s.e.m. of three independent experiments. Analysis was performed with one-way ANOVA followed by Tukey–Kramer post hoc analysis. * P <0.05 versus H 2 O 2 alone. ( d ) miR-421 is upregulated in response to I/R injury. Mice were subjected to I/R as described in Methods. MiR-421 levels were detected by qRT–PCR. Data are shown as mean±s.e.m. of five independent experiments. * P <0.05 versus sham in Student’s t -test. ( e , f ) Knockdown of miR-421 attenuates mitochondrial fragmentation on I/R. Adult male C57BL/6 mice (8 weeks old) were delivered in 3 consecutive days, intravenous injections of miR-421 antagomir (anta-421) or antagomir control (anta-NC) at doses of 30 mg kg −1 body weight. Three days after injection, the mice were subjected to I/R. The fragmented mitochondria were shown in e and counting of the fragmented mitochondria was shown in f . Data are shown as mean±s.e.m. of six independent experiments. Analysis was performed with one-way ANOVA followed by Tukey–Kramer post hoc analysis. * P <0.05 versus I/R alone. ( g ) Knockdown of miR-421 attenuates apoptosis on I/R. Counting of the apoptotic cell was shown. TUNEL-positive cardiomyocyte nuclei (apoptotic cells) were green. Nuclei stained by DAPI showed blue. Cardiomyocytes were labelled with α-actinin. Data are shown as mean±s.e.m. of six independent experiments. Analysis was performed with one-way ANOVA followed by Tukey–Kramer post hoc analysis. * P <0.05 versus I/R alone. DAPI, 4,6-diamidino-2-phenylindole. Full size image Subsequently, we detected whether miR-421 was involved in the pathogenesis of myocardial infarction in the animal model. MiR-421 was elevated in response to I/R injury ( Fig. 3d ). Knockdown of miR-421 by antagomir delivery in vivo ( Supplementary Fig. 7a ) resulted in a reduction in mitochondrial fragmentation ( Fig. 3e,f ) and apoptosis ( Fig. 3g ). The cardiac function was ameliorated in the miR-421-knockdown group ( Supplementary Fig. 7b ). In addition, we also demonstrated that enforced expression of miR-421 in cardiomyocytes induced mitochondrial fragmentation and apoptosis, and Pink1-TP miR-421 attenuated the effect of miR-421 on mitochondrial fragmentation and apoptosis ( Supplementary Fig. 7c,d ), indicating that miR-421-regulated mitochondrial fragmentation and apoptosis via Pink1. miR-421-transgenic mice potentiate myocardial infarction In animal model, we generated miR-421-transgenic mice ( Fig. 4a–c ) and found that miR-421-transgenic mice potentiated mitochondrial fragmentation and apoptosis on I/R injury ( Fig. 4d,e ;). MiR-421-transgenic mice also showed an enlarged myocardial infarct sizes, compared with the WT group in response to I/R ( Fig. 4f ). These data suggest that miR-421 participates in mediating the signal for mitochondrial fragmentation and apoptosis in the heart. 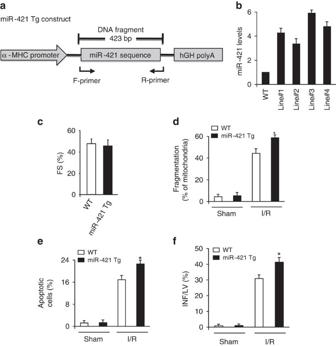Figure 4: miR-421-transgenic mice potentiate myocardial infarction. (a) Schematic map showing the transgenic construct of miR-421. (b) Detection of miR-421 levels in miR-421-transgenic mice. The expression of miR-421 was analysed by qRT–PCR from wild type (WT) and different lines of miR-421-transgenic mice. (c) miR-421-transgenic mice developed normally without obvious cardiac function alterations under basal conditions. Fractional shortening (FS) was shown. (n=8 per group). (d–f) miR-421-transgenic mice exhibited increased mitochondrial fragmentation, apoptosis and myocardial infarction sizes in response to I/R. WT C57BL/6 mice and miR-421-transgenic mice (8 weeks old) were subjected to I/R. Mitochondrial fragmentation (d), apoptosis (e) and myocardial infarction sizes (f) were analysed. Data are shown as mean±s.e.m. of eight independent experiments. Analysis was performed with one-way analysis of variance followed by Tukey–Kramerpost hocanalysis. *P<0.05 versus WT+I/R. Figure 4: miR-421-transgenic mice potentiate myocardial infarction. ( a ) Schematic map showing the transgenic construct of miR-421. ( b ) Detection of miR-421 levels in miR-421-transgenic mice. The expression of miR-421 was analysed by qRT–PCR from wild type (WT) and different lines of miR-421-transgenic mice. ( c ) miR-421-transgenic mice developed normally without obvious cardiac function alterations under basal conditions. Fractional shortening (FS) was shown. ( n =8 per group). ( d – f ) miR-421-transgenic mice exhibited increased mitochondrial fragmentation, apoptosis and myocardial infarction sizes in response to I/R. WT C57BL/6 mice and miR-421-transgenic mice (8 weeks old) were subjected to I/R. Mitochondrial fragmentation ( d ), apoptosis ( e ) and myocardial infarction sizes ( f ) were analysed. Data are shown as mean±s.e.m. of eight independent experiments. Analysis was performed with one-way analysis of variance followed by Tukey–Kramer post hoc analysis. * P <0.05 versus WT+I/R. Full size image miR-421 exerts its function through targeting Pink1 We explored how miR-421 exerted its effect on mitochondrial fragmentation and apoptotic program. As miR-421 was able to suppress Pink1 expression, we thus tested whether Pink1 was a downstream mediator of miR-421. SiRNA-induced gene silencing could significantly reduce Pink1 expression levels ( Fig. 5a ). Knockdown of miR-421 inhibited the decrease of Pink1, mitochondrial fragmentation and apoptosis, which are induced by H 2 O 2 . However, the inhibitory effect of miR-421 downregulation was attenuated by Pink1 knockdown ( Fig. 5b,c ). Our results also further showed that the target protector of Pink1 inhibited mitochondrial fragmentation ( Fig. 5d ) and apoptosis ( Fig. 5e ) induced by H 2 O 2 . These data suggest that miR-421 and Pink1 are functionally linked and miR-421 targets Pink1 in the signalling cascades of mitochondrial fragmentation and apoptosis in cardiomyocytes. 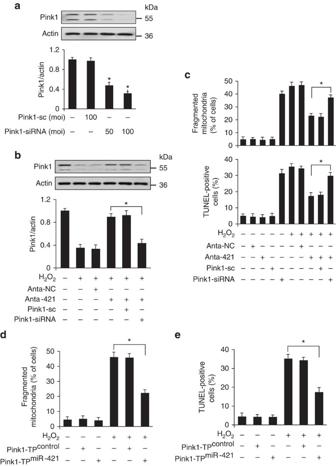Figure 5: miR-421 regulates mitochondrial dynamics and apoptosis by Pink1. (a) Expression of Pink1 is knocked down by siRNA-mediated gene silencing. Cardiomyocytes were infected with adenoviral Pink1-siRNA or its scramble form (Pink1-sc) at the indicated moi. Pink1 levels were detected by immunoblot. Quantitative analysis of expression levels of Pink1 protein were shown in lower panel. Data are shown as mean±s.e.m. of three independent experiments. *P<0.05 versus untreated group in Student’st-test. (b,c) Knockdown of Pink1 attenuates the inhibitory effect of miR-421 antagomir on mitochondrial fragmentation and apoptosis on H2O2. Cardiomyocytes were infected with adenoviral Pink1-siRNA or its scramble form, transfected with anta-421 or anta-NC, and then exposed to H2O2. Cells were harvested for the analysis of Pink1 expression levels (b), mitochondrial fragmentation (c, upper panel) and apoptosis (c, low panel). Data are shown as mean±s.e.m. of three independent experiments. Analysis was performed with one-way analysis of variance (ANOVA) followed by Tukey–Kramerpost hocanalysis. *P<0.05. (d,e) Pink1 target protector inhibits mitochondrial fragmentation and apoptosis induced by H2O2. Cardiomyocytes were transfected with the target protector (Pink1-TPmiR-421) or the control (Pink1-TPcontrol), and then exposed to H2O2. Mitochondrial fragmentation (d) and apoptosis (e) were analysed. Data are shown as mean±s.e.m. of four independent experiments. Analysis was performed with one-way ANOVA followed by Tukey–Kramerpost hocanalysis. *P<0.05. Figure 5: miR-421 regulates mitochondrial dynamics and apoptosis by Pink1. ( a ) Expression of Pink1 is knocked down by siRNA-mediated gene silencing. Cardiomyocytes were infected with adenoviral Pink1-siRNA or its scramble form (Pink1-sc) at the indicated moi. Pink1 levels were detected by immunoblot. Quantitative analysis of expression levels of Pink1 protein were shown in lower panel. Data are shown as mean±s.e.m. of three independent experiments. * P <0.05 versus untreated group in Student’s t -test. ( b , c ) Knockdown of Pink1 attenuates the inhibitory effect of miR-421 antagomir on mitochondrial fragmentation and apoptosis on H 2 O 2 . Cardiomyocytes were infected with adenoviral Pink1-siRNA or its scramble form, transfected with anta-421 or anta-NC, and then exposed to H 2 O 2 . Cells were harvested for the analysis of Pink1 expression levels ( b ), mitochondrial fragmentation ( c , upper panel) and apoptosis ( c , low panel). Data are shown as mean±s.e.m. of three independent experiments. Analysis was performed with one-way analysis of variance (ANOVA) followed by Tukey–Kramer post hoc analysis. * P <0.05. ( d , e ) Pink1 target protector inhibits mitochondrial fragmentation and apoptosis induced by H 2 O 2 . Cardiomyocytes were transfected with the target protector (Pink1-TP miR-421 ) or the control (Pink1-TP control ), and then exposed to H 2 O 2 . Mitochondrial fragmentation ( d ) and apoptosis ( e ) were analysed. Data are shown as mean±s.e.m. of four independent experiments. Analysis was performed with one-way ANOVA followed by Tukey–Kramer post hoc analysis. * P <0.05. Full size image We also produced miR-421/Pink1-bitransgenic mice (miR-421/Pink1), and miR-421/Pink1-bitransgenic mice exhibited a reduced mitochondrial fragmentation ( Supplementary Fig. 8a ), apoptosis ( Supplementary Fig. 8b ) and myocardial infarct sizes ( Supplementary Fig. 8c ) compared with miR-421-transgenic mice alone on I/R injury, suggesting that miR-421 and Pink1 had a cross-talk in the animal model. E2F1 activates miR-421 transcription We asked how miR-421 expression is regulated under the pathological condition. Our previous work had shown that the expression of miRNA could be regulated at the transcriptional level. Thus, we analysed the promoter region of mouse miR-421 and observed that there was a potential binding site of E2F1 ( Fig. 6a ). We further tested whether E2F1 could influence miR-421 promoter activity. The luciferase assay demonstrated that E2F1 stimulated the wild-type (WT) miR-421 promoter activity ( Fig. 6b ). However, mutations in the E2F1-binding site abolished the effect of E2F1 on miR-421 promoter activity ( Fig. 6b ). Enforced expression of E2F1 led to an increase of miR-421 levels ( Fig. 6c ), whereas E2F1 KO mice exhibited a decreased expression levels of miR-421 ( Fig. 6d ). Next, we tested whether E2F1 could bind to the promoter region of miR-421. The chromatin immunoprecipitation (ChIP) assay revealed that E2F1 bound to the miR-421 promoter under the physiological condition. H 2 O 2 treatment led to an increase in the association levels of E2F1 with miR-421 promoter ( Fig. 6e ), suggesting that miR-421 is a potential transcriptional target of E2F1. Furthermore, H 2 O 2 induced an elevation in miR-421 promoter activity in cardiomyocytes ( Fig. 6f ), and knockdown of E2F1 attenuated the increase of miR-421 promoter activity induced by H 2 O 2 ( Fig. 6f ). These data indicate that miR-421 can be transcriptionally activated by E2F1. 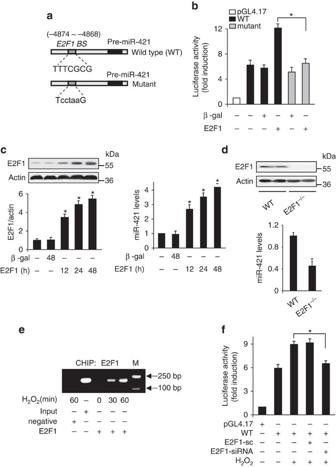Figure 6: miR-421 is a transcriptional target of E2F1. (a) Mouse miR-421 promoter region contains a potential E2F1-binding site. (b) E2F1 activates miR-421 promoter activity. Cardiomyocytes were treated with the adenoviral β-gal or E2F1, the constructs of the empty vector (pGL-4.17), the wild type promoter or the promoter with mutations in the binding site (mutant), respectively. Luciferase activity was assayed. Data are shown as mean±s.e.m. of four independent experiments. Analysis was performed with one-way analysis of variance (ANOVA) followed by Tukey–Kramerpost hocanalysis. *P<0.05. (c) E2F1 promotes miR-421 expression. Cardiomyocytes were infected with adenoviral β-gal or E2F1. E2F1 expression was analysed by immunoblot (left panel). Quantitative analysis of expression levels of E2F1 protein shown in lower panel. MiR-421 levels were analysed by qRT–PCR (right panel). Data are shown as mean±s.e.m. of four independent experiments. *P<0.05 versus untreated group in Student’st-test. (d) MiR-421 levels in E2F1-deficient mice. E2F1-knockout mice (KO), wild-type littermates (WT). Data are shown as mean±s.e.m. of six independent experiments. *P<0.05 versus WT in Student’st-test. (e) ChIP analysis of E2F1 binding to the promoter of miR-421. (f) Knockdown of E2F1 attenuates the increase of miR-421 promoter activity induced by H2O2. Cardiomyocytes were treated with the adenoviral E2F1-siRNA or E2F1-sc, the constructs of the empty vector (pGL-4.17), the wild type (WT) promoter, then were treated with H2O2. Luciferase activity was assayed. Data are shown as mean±s.e.m. of three independent experiments. Analysis was performed with one-way ANOVA followed by Tukey–Kramerpost hocanalysis. *P<0.05. Figure 6: miR-421 is a transcriptional target of E2F1. ( a ) Mouse miR-421 promoter region contains a potential E2F1-binding site. ( b ) E2F1 activates miR-421 promoter activity. Cardiomyocytes were treated with the adenoviral β-gal or E2F1, the constructs of the empty vector (pGL-4.17), the wild type promoter or the promoter with mutations in the binding site (mutant), respectively. Luciferase activity was assayed. Data are shown as mean±s.e.m. of four independent experiments. Analysis was performed with one-way analysis of variance (ANOVA) followed by Tukey–Kramer post hoc analysis. * P <0.05. ( c ) E2F1 promotes miR-421 expression. Cardiomyocytes were infected with adenoviral β-gal or E2F1. E2F1 expression was analysed by immunoblot (left panel). Quantitative analysis of expression levels of E2F1 protein shown in lower panel. MiR-421 levels were analysed by qRT–PCR (right panel). Data are shown as mean±s.e.m. of four independent experiments. * P <0.05 versus untreated group in Student’s t -test. ( d ) MiR-421 levels in E2F1-deficient mice. E2F1-knockout mice (KO), wild-type littermates (WT). Data are shown as mean±s.e.m. of six independent experiments. * P <0.05 versus WT in Student’s t -test. ( e ) ChIP analysis of E2F1 binding to the promoter of miR-421. ( f ) Knockdown of E2F1 attenuates the increase of miR-421 promoter activity induced by H 2 O 2 . Cardiomyocytes were treated with the adenoviral E2F1-siRNA or E2F1-sc, the constructs of the empty vector (pGL-4.17), the wild type (WT) promoter, then were treated with H 2 O 2 . Luciferase activity was assayed. Data are shown as mean±s.e.m. of three independent experiments. Analysis was performed with one-way ANOVA followed by Tukey–Kramer post hoc analysis. * P <0.05. Full size image E2F1 regulates mitochondrial dynamics by miR-421 and Pink1 We investigated the role of E2F1 in mitochondrial fragmentation and apoptosis in cardiomyocytes and myocardial infarction. H 2 O 2 induced an elevation in E2F1 expression level ( Fig. 7a ). Enforced expression of E2F1 provoked mitochondrial fragmentation ( Fig. 7b ) and apoptosis ( Fig. 7c ). Knockdown of E2F1 was able to attenuate E2F1 expression ( Fig. 7d ), mitochondrial fragmentation ( Fig. 7e , upper panel) and apoptosis ( Fig. 7e , lower panel) on H 2 O 2 . Furthermore, E2F1 KO mice demonstrated reduced mitochondrial fragmentation ( Fig. 7f ), apoptosis ( Fig. 7g ) and myocardial infarction size ( Fig. 7h ) on I/R injury. The cardiac function was also ameliorated in the E2F1 KO mice group ( Supplementary Fig. 9 ). These data suggest that E2F1 participates in mediating the signal for mitochondrial fragmentation and apoptosis in the heart. 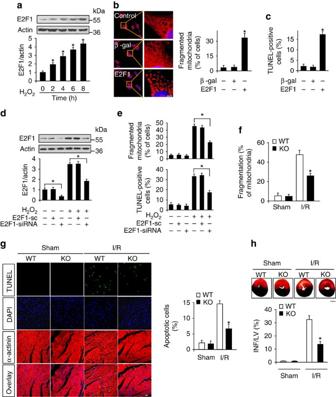Figure 7: E2F1 promotes mitochondrial fragmentation and apoptosis. (a) Cardiomyocytes were exposed to H2O2. Cells were harvested at the indicated time for the analysis of E2F1 levels by immunoblot. Data are shown as mean±s.e.m. of three independent experiments. *P<0.05 versus untreated group in Student’st-test. (b,c) Enforced expression of E2F1 induces mitochondrial fragmentation and apoptosis. Cardiomyocytes were infected with adenoviral E2F1 or β-gal. Forty-eight hours after infection mitochondrial fragmentation (b) and apoptosis (c) were analysed. Data are shown as mean±s.e.m. of three independent experiments. Analysis was performed with one-way analysis of variance (ANOVA) followed by Tukey–Kramerpost hocanalysis. *P<0.05 versus untreated group. (d) Cardiomyocytes were infected with adenoviral E2F1-siRNA or E2F1-sc, and then exposed to H2O2. E2F1 levels were detected by immunoblot. Data are shown as mean±s.e.m. of three independent experiments. Analysis was performed with one-way ANOVA followed by Tukey–Kramerpost hocanalysis. *P<0.05. (e) Knockdown of E2F1 reduces mitochondrial fragmentation and apoptosis. Cardiomyocytes were treated as described ind, mitochondrial fragmentation (upper panel) and apoptosis (lower panel) were analysed. Data are shown as mean±s.e.m. of three independent experiments. Analysis was performed with one-way ANOVA followed by Tukey–Kramerpost hocanalysis. *P<0.05. (f,g) E2F1-knockout mice attenuates mitochondrial fragmentation and apoptosis on I/R. WT and E2F1-knockout mice were subjected to I/R as described in Methods. Mitochondrial fragmentation (f) and apoptosis (g) were analysed. Data are shown as mean±s.e.m. of six independent experiments. Analysis was performed with one-way ANOVA followed by Tukey–Kramerpost hocanalysis. *P<0.05 versus WT+I/R. (h) E2F1-knockout mice attenuates myocardial infarction sizes on I/R. WT and E2F1-knockout mice were subjected to I/R as described inf. The upper panels are representative photos of midventricular myocardial slices. The lower panel shows infarct sizes. Data are shown as mean±s.e.m. of six independent experiments. Analysis was performed with one-way ANOVA followed by Tukey–Kramerpost hocanalysis. *P<0.05 versus WT+I/R. Bar=2 mm. Figure 7: E2F1 promotes mitochondrial fragmentation and apoptosis. ( a ) Cardiomyocytes were exposed to H 2 O 2 . Cells were harvested at the indicated time for the analysis of E2F1 levels by immunoblot. Data are shown as mean±s.e.m. of three independent experiments. * P <0.05 versus untreated group in Student’s t -test. ( b , c ) Enforced expression of E2F1 induces mitochondrial fragmentation and apoptosis. Cardiomyocytes were infected with adenoviral E2F1 or β-gal. Forty-eight hours after infection mitochondrial fragmentation ( b ) and apoptosis ( c ) were analysed. Data are shown as mean±s.e.m. of three independent experiments. Analysis was performed with one-way analysis of variance (ANOVA) followed by Tukey–Kramer post hoc analysis. * P <0.05 versus untreated group. ( d ) Cardiomyocytes were infected with adenoviral E2F1-siRNA or E2F1-sc, and then exposed to H 2 O 2 . E2F1 levels were detected by immunoblot. Data are shown as mean±s.e.m. of three independent experiments. Analysis was performed with one-way ANOVA followed by Tukey–Kramer post hoc analysis. * P <0.05. ( e ) Knockdown of E2F1 reduces mitochondrial fragmentation and apoptosis. Cardiomyocytes were treated as described in d , mitochondrial fragmentation (upper panel) and apoptosis (lower panel) were analysed. Data are shown as mean±s.e.m. of three independent experiments. Analysis was performed with one-way ANOVA followed by Tukey–Kramer post hoc analysis. * P <0.05. ( f , g ) E2F1-knockout mice attenuates mitochondrial fragmentation and apoptosis on I/R. WT and E2F1-knockout mice were subjected to I/R as described in Methods. Mitochondrial fragmentation ( f ) and apoptosis ( g ) were analysed. Data are shown as mean±s.e.m. of six independent experiments. Analysis was performed with one-way ANOVA followed by Tukey–Kramer post hoc analysis. * P <0.05 versus WT+I/R. ( h ) E2F1-knockout mice attenuates myocardial infarction sizes on I/R. WT and E2F1-knockout mice were subjected to I/R as described in f . The upper panels are representative photos of midventricular myocardial slices. The lower panel shows infarct sizes. Data are shown as mean±s.e.m. of six independent experiments. Analysis was performed with one-way ANOVA followed by Tukey–Kramer post hoc analysis. * P <0.05 versus WT+I/R. Bar=2 mm. Full size image We further explored whether Pink1 could act as the downstream target of E2F1 in mitochondrial regulatory signal pathway. We observed that the knockdown of Pink1 attenuated the effect of E2F1 knockdown on Pink1 expression ( Supplementary Fig. 10a ), mitochondrial fragmentation ( Supplementary Fig. 10b , upper panel) and apoptosis ( Supplementary Fig. 10b , lower panel) in response to H 2 O 2 . Taken together, E2F1, miR-421 and Pink1 constitute an axis in regulating mitochondrial dynamics and apoptosis in the heart. Mitochondria are enriched in cardiomyocytes and are essential for cardiomyocytes function. Dysfunction in mitochondria usually results in deficit in cardiac energetic metabolism and increased oxidative stress, which are all critical components contribute to cardiac disorders including myocardial infarction and heart failure [6] , [7] . Thus, it is necessary to elucidate the molecular mechanisms of mitochondrial regulation, and discover potential therapeutic targets for inhibiting myocardial infarction and the consequent heart failure. Our present work demonstrates that Pink1 can inhibit mitochondrial fragmentation and apoptosis in cardiomyocytes and reduce myocardial infarction in the animal model. In addition, we demonstrate that miR-421 is responsible for the downregulation of Pink1, and modulation of miR-421 levels also affects mitochondrial fragmentation, apoptosis and myocardial infarction. MiR-421 exerts its effect on mitochondrial fragmentation and apoptosis in a Pink1-dependent manner. We further identify that E2F1 regulates mitochondrial fragmentation and apoptosis through targeting miR-421 in transcriptional level. Our results provide novel evidence demonstrating that E2F1, miR-421 and Pink1 constitute an axis in the regulated machinery of mitochondrial network. The regulation of their levels provides therapeutic targets for treating myocardial infarction and heart failure. The present work shows that Pink1 is able to inhibit mitochondrial fragmentation. This is in consistence with other reports that demonstrate the protective effect of Pink1 on mitochondrial integrity. For example, Pink1 is mutated in parkinsonism, and overexpression of the WT Pink1, but not the parkinsonism-associated mutant, protects cells from apoptosis in response to oxidative stress [25] , [33] . Inhibition of Pink1 induces fragmented mitochondria, altered cristae morphology and reduced membrane potential [34] . Overexpression of Pink1 rescues mitochondrial fragmentation [35] , increases mitochondrial interconnectivity [12] and reduces mitochondrial dysfunction and apoptosis as well [36] . Our present study for the first time reveals that Pink1 can maintain the cardiac structure and function through its protective effect on the mitochondria. Our results may have important therapeutic implications for the employment of Pink1 in the treatment of apoptosis-related cardiac diseases. Accumulating studies have shown that mitochondrial fragmentation is required for the induction of apoptosis. For example, knockdown of Drp1 inhibits mitochondrial fragmentation and p53-dependent apoptosis [7] , [37] . Enforced expression of Mfn2 leads to mitochondrial fusion that is important for cell survival [38] . Our present work demonstrates that Pink1 is able to inhibit mitochondrial fragmentation and the consequent apoptosis. This result supports the notion that mitochondrial fragmentation and apoptosis are two linked events. However, there are reports showing that mitochondrial dynamics is not invariably related to apoptosis. For instance, downregulation of Drp1 partially inhibits the release of cytochrome c , but does not inhibit the release of Smac/DIABLO. Subsequently, it only delays but not inhibits apoptosis [39] . Overexpression of OPA1 does not protect ischaemia-induced apoptosis, although it alters mitochondrial dynamics [40] . Such a discrepancy may be due to the expression patterns of apoptotic factors and the molecules regulating mitochondrial network in different cell types. MiRNAs participate in various biological and pathological processes, such as apoptosis, development and proliferation. Some miRNAs have been reported to regulate apoptosis in cardiomyocytes [6] , [41] , [42] . However, few works have been focused on miRNAs in the mitochondrial network regulation. It is critical to identify those miRNAs that can regulate mitochondrial dynamics and apoptosis in the heart and to characterize their signal transduction pathways in the apoptotic cascades. Previous studies have shown that miR-421 has an important functional role in multiple cancer cell types [43] , [44] , [45] , [46] , [47] . Our present work for the first time demonstrates that miR-421 is able to regulate mitochondrial fragmentation and apoptosis both in vitro and in vivo through targeting Pink1. Available researches consistently suggest that miRNA modulations can be promising and fascinating therapies in heart diseases and our work identifies miR-421 as a potential therapeutic target. Emerging evidences suggest that E2Fs function in a wide range of biological processes, including DNA replication, mitosis, the mitotic checkpoint, DNA damage checkpoints, DNA repair, differentiation and development [48] . The mechanism of E2F1 in inducing apoptosis has been widely studied [49] . However, E2F1 function in the regulation of mitochondrial dynamics in apoptotic signalling pathway remains unknown. In present work, we demonstrate that an important, and hitherto unrecognized, feature of E2F1 function is the regulation of mitochondrial fragmentation. Our results show that knockdown of E2F1 inhibits mitochondrial fragmentation and apoptosis in cardiomyocytes. E2F1 KO mice demonstrate reduced mitochondrial fragmentation and myocardial infarction size on I/R injury. E2F1 participates in the mitochondrial network and apoptotic pathway by regulating the expression of miR-421. It would be interesting to study the role of other E2F1 targets in the cascades of mitochondrial network. Modulation of their levels may provide a new approach for tackling myocardial infarction. Generation of cardiac-specific-transgenic mice For creating miR-421-transgenic mice, a DNA fragment containing murine miR-421 was cloned in the vector pαMHC-clone26 (kindly provided by Dr. Zhong Zhou Yang), under the control of the α-myosin heavy chain (α-MHC) promoter. The primers used to generate miR-421-transgenic mice were the following: forward primer 5′-AAACTAATCCGTAAGGGCAA-3′; reverse primer 5′-ACACAGGCATAAATACAGTA-3′. For generation of Pink1-transgenic mice, the mouse Pink1-coding sequence was synthesized by PCR using mouse complementary DNA (cDNA) as the template and was cloned into the vector pαMHC-clone26 under the control of the α-MHC promoter. The primers used to generate Pink1-transgenic mice included, forward primer: 5′-CGCCACCATGGCGGTGCGACAGG-3′; reverse primer: 5′-CATGGGGCTGCCCTCCAGGAAG-3′. Microinjection was performed following standard protocols. E2F1-knockout mice E2F1 KO mice were purchased from Mutant Mouse Regional Resource Center, USA. E2F1 +/− mice were interbred to give KO mice (E2F1 −/− ), which were used for further studies. Mice were genotyped by multiplex PCR (primers and conditions are available from Mutant Mouse Regional Resource Center, USA). All experiments were performed on E2F1 −/− mice and their WT littermates (E2F1 +/+ ). The animal experiments were performed according to the protocols approved by the Institute Animal Care Committee and were approved by government authorities. Cardiomyocyte culture and treatment Cardiomyocytes were isolated from male mice (1–2 days), which were obtained from Institute of Laboratory Animal Science of Chinese Academy of Medical Sciences (Beijing, China). Briefly, after dissection, the hearts were washed and minced in HEPES-buffered saline solution. Tissues were then dispersed in a series of incubations at 37 °C in HEPES-buffered saline solution containing 1.2 mg ml −1 pancreatin and 0.14 mg ml −1 collagenase. Subsequent supernatants were collected and centrifuged at 200 g for 5 min. After centrifugation, cells were resuspended in Dulbecco’s modified Eagle medium/F-12 (Gibco) containing 5% heat-inactivated horse serum, 0.1 mM ascorbate, insulin-transferrin-sodium selenite media supplement (Sigma, St Louis, MO), 100 U ml −1 penicillin, 100 μg ml −1 streptomycin and 0.1 mM bromodeoxyuridine. The dissociated cells were pre-plated at 37 °C for 1 h. The cells were then diluted to 1 × 10 6 cells per ml and plated in 10 μg ml −1 laminin-coated different culture dishes according to the specific experimental requirements. Cells were treated with 150 μM H 2 O 2 for the indicated periods of time. Apoptosis assays Apoptosis was determined by the terminal deoxyribonucleotidyl transferase-mediated TdT-mediated dUTP nick end labelling using a kit from Roche. The detection procedures were in accordance with the kit instructions. Preparations of miR-421 expression constructs miR-421 was synthesized by PCR using mouse genomic DNA as the template. The upstream primer was 5′-TGGAGTGGTGTTCCTCTGAAGAAAT-3′; the downstream primer was 5′-TAGAAAAGAACCAGATATGGAATCC-3′. The generated PCR fragment was cloned into the Adeno-X T Expression System (Clontech), according to the manufacturer’s instructions. Adenoviral constructions and infection The mouse Pink1 cDNA was synthesized by PCR using mouse cDNA as the template. Mouse E2F1 cDNA was purchased from Origene. The adenoviruses harbouring Pink1 and E2F1 were constructed using the Adeno-X expression system (Clontech). The mouse Pink1 RNA interference (siRNA) target sequence is 5′-CCAAGCGCGTGTCTGACCC-3′. A scramble form was used as a control, 5′-AGCCGTCGACTGCACTCGC-3′. E2F1 siRNA sequence is 5′-ATCTGACCACCAAACGCTT-3′; the scramble E2F1 siRNA sequence is 5′-CACTCACGACTACGATCTA-3′. TRAP1 siRNA sequence is 5′-GGAGGAGGAGAGCCTGCAC-3′; the scramble TRAP1 siRNA sequence is 5′-GAGGACTGACAGGCAGCGG-3′. The adenoviruses harbouring siRNAs or their scramble forms were constructed using the pSilencer adeno 1.0-CMV System (Ambion) according to the Kit’s instructions. All constructs were amplified in HEK293 cells. HEK293 cells (CRL-1573) are purchased from the American Type Culture Collection and cultured in DMEM containing 10% FBS (Invitrogen). Transfection of the antagomir The chemically modified antagomir complementary to miR-421 that was designed to inhibit endogenous miR-421 expression and the antagomir negative control (antagomir-NC) were obtained from GenePharma Co. Ltd. The miR-421 antagomir sequence was 5′-AUUCAACAAACAUUUAAUGAG-3′. The antagomir-NC sequence was 5′-CAGUACUUUUGUGUAGUACAA-3′. Cardiomyocytes were transfected with the miR-421 antagomir or the antagomir-NC using Lipofectamine 2000 (Invitrogen) according to the manufacturer’s instruction. Target protector preparation and transfection Target protector was designed to disrupt the interaction of specific miRNA–mRNA pairs. Target protector sequence is complementary to miR-421-binding site in target Pink1. In brief, Pink1-TP miR-421 sequence was 5′-GGCCTCACTGCAGTGCTTGCTTGGC-3′. Pink1-TP control sequence was 5′-TGACAAATGAGACTCTCTCCTCTCC-3′. They were synthesized by Gene Tools, and were transfected into the cells using the Endo-Porter kit (Gene Tools) according to the kit’s instructions. Immunoblot Immunoblot was performed as follows. The cells were lysed for 1 h at 4 °C in a lysis buffer (20 mmol l −1 Tris pH 7.5, 2 mmol l −1 EDTA, 3 mmol l −1 EGTA, 2 mmol l −1 dithiothreitol (DTT), 250 mmol l −1 sucrose, 0.1 mmol l −1 phenylmethylsulfonyl fluoride and 1% Triton X-100) containing a protease inhibitor cocktail. The samples were subjected to 12% SDS–polyacrylamide gel electrophoresis and transferred to nitrocellulose membranes. Equal protein loading was controlled by Ponceau Red staining of membranes. Blots were probed using the primary antibodies. The anti-Pink1 (1:500), anti-Parkin (1:500), anti-Cox IV (1:1,000), anti-E2F1 (1:1,000), anti-Miro (1:1,000), anti-Mfn2 (1:500), anti-Phosphoserine (1:500) and anti-beta actin (1:2,000) were from Abcam. The anti-Drp1 (1:1,000) was from BD Biosciences. The anti-tubulin (1:2,000) and anti-TRAP1 (1:1,000) were from Santa Cruz Biotechnology. After four times washing with PBS, the horseradish peroxidase-conjugated goat anti-rabbit IgG (1:2,000) or rabbit anti-goat IgG (1:2,000) were purchased from Santa Cruz Biotechnology. Antigen–antibody complexes were visualized by enhanced chemiluminescence. Full-sized scans of western blots are provided in Supplementary Figs 11 and 12 . Quantitative real-time PCR Stem-loop qRT–PCR for mature miR-421 was performed on a CFX96 Real-Time PCR Detection System (Bio-Rad). Total RNA was extracted using Trizol reagent. After DNAse I (Takara, Japan) treatment, RNA was reverse transcribed with reverse transcriptase (ReverTra Ace, Toyobo). The levels of miR-421 analysed by qRT–PCR were normalized to that of U6. MiR-421 primers were forward: 5′-ATCAACAGACATTAATTGGGC-3′; reverse: 5′-GTGCAGGGTCCGAGGT-3′. U6 primers were forward: 5′-GCTTCGGCAGCACATATACT-3′; reverse: 5′-AACGCTTCACGAATTTGCGT-3′. Absolute quantification using qRT–PCR We measured the absolute copy number using the standard curve method. Synthetic miR-421 RNA was used as the standard of miR-421. For detection of miR-421, the standard of miR-421 was reverse transcribed the same as endogenous miR-421. The standard cDNA was serially diluted in nuclease-free water. Serial dilutions from 10 6 to 10 1 copies were used for standard in a final volume of 20 μl alongside a negative control (RNA) and a non-template control. The SYBR Premix Ex Taq II Kit (Takara) was used for amplification. Quantitative PCR was performed on a CFX96 Real-Time PCR Detection System (Bio-Rad). Absolute quantification determines the actual copy numbers of target genes by relating the Ct value to a standard curve. The data were analysed by CFX96 software. The final data were expressed as the copy number per 10 pg of total RNA. Luciferase activity assay Pink1 3′-UTR was amplified by PCR. The forward primer was 5′-GTGCTCCAGTTACTAAAAGAC-3′; the reverse primer was 5′-TTGACTATGAGCCATGCTGG-3′. To produce mutated 3′-UTR, the mutations were generated using QuikChange II XL Site-Directed Mutagenesis Kit (Stratagene). The constructs were sequence verified. WT and mutated 3′-UTRs were subcloned into the pGL3 vector (Promega) immediately downstream of the stop codon of the luciferase gene. Luciferase activity assay was performed using the Dual-Luciferase Reporter Assay System (Promega) according to the manufacturer’s instructions. Cells were co-transfected with the plasmid constructs of 150 ng per well of pGL3-Pink1-3′-UTR or pGL3-Pink1-3′-UTR-mut using Lipofectamine 2000 (Invitrogen), then were infected with adenovirus miR-421 or β-gal at a moi of 80. At 48 h after infection, luciferase activity was measured. Constructions of mouse miR-421 promoter and its mutant The promoter of miR-421 was amplified from mouse genome using PCR. The forward primer was 5′-GTATGTATGTATGTATGTATGTATG-3′. The reverse primer was 5′-TCTGTCATTAAATAAAGCTCAC-3′. The promoter fragment was finally cloned into the vector pGL4.17 (Promega). The introduction of mutations in the putative E2F1-binding site was performed with the QuikChange II XL Site-Directed Mutagenesis Kit (Stratagene) using the WT vector as a template. The construct was sequenced to check that only the desired mutations had been introduced. Chromatin immunoprecipitation assay ChIP assay was performed as follows. Cells were washed with PBS and incubated for 10 min with 1% formaldehyde at room temperature. The cross-linking was quenched with 0.1 M glycine for 5 min. Cells were washed twice with PBS and lysed for 1 h at 4 °C in a lysis buffer. The cell lysates were sonicated into chromatin fragments with an average length of 500–800 bp as assessed by agarose gel electrophoresis. The samples were precleared with Protein-A agarose (Roche) for 1 h at 4 °C on a rocking platform, and 5 μg specific antibodies were added and rocked for overnight at 4 °C. Immunoprecipitates were captured with 10% (vol/vol) Protein-A agarose for 4 h. Before use, Protein-A agarose was blocked twice at 4 °C with salmon sperm DNA (2 μg ml −1 ) overnight. DNA fragments were purified with a QIAquick Spin Kit (Qiagen). The purified DNA was used as a template and amplified with the following primer sets: for the analysis of E2F1 binding to the promoter region of miR-421, the oligonucleotides were as follows: forward: 5′-GTATGTATGTATGTATGTATGTATG-3′; reverse: 5′-GAGCAAAATAGGACATAGC-3′. Mitochondrial staining Mitochondrial staining was carried as follows. Cells were plated onto the cover slips coated with 0.01% poly- L -lysine. After treatment, they were stained for 20 min with 0.02 μM MitoTracker Red CMXRos (Molecular Probes). Mitochondria were imaged using a laser scanning confocal microscope (Zeiss LSM510 META). The percentage of cells with fragmented mitochondria relative to the total number of cells was presented as the mean±s.e.m. of at least three independent experiments, counted by an observer blinded to the experimental conditions. Six distinct fields for each 50 cells were counted. At least 300 cells per group were counted. Electron microscopy Heart ultrastructural analyses were performed to quantify mitochondrial fragmentation. Samples were examined at a magnification of 15,000 with a JEOL JEM-1230 transmission electron microscope. For comparison of mitochondrial fragmentation, electron microscope micrographs of thin sections were evaluated. The size of individual mitochondrion was measured using Image-Pro Plus software. Approximately 1,200–1,500 mitochondria were measured to determine the percentages of mitochondria with various sizes. In I/R-treated heart tissues, mitochondria disintegrated into numerous small round fragments of varying size, the number of small mitochondrion was increasing. Thus, we determined the mitochondria with size <0.6 mm 2 as fragmentation mitochondria. For fusion mitochondria, the proportions of interfibrillar mitochondria with lengths that were >2 μm (the length of a single sarcomere) were determined. Measurement of cardiac mitochondrial ATP levels Hearts were collected from control and Pink1-transgenic mice, and homogenized in ice-cold homogenization solution. Mitochondria were isolated and cardiac mitochondrial ATP levels were measured using a luciferase-based ATP determination kit (Molecular Probes). ATP assays were performed on 10 μl of resuspended mitochondria, and each sample was measured in triplicate. Animal experiments Male adult C57BL/6 mice (8 weeks old) were obtained from Institute of Laboratory Animal Science of Chinese Academy of Medical Sciences (Beijing, China). All experiments were performed according to the protocols approved by the Institute Animal Care Committee, Qingdao University. The animals we chose for experiments had similar body weight. And animals with normal physiological index during surgical experiments were used for statistical analysis. For miR-421 antagomir delivery, the mice received on 3 consecutive days, intravenous injections of miR-421 antagomir, or its control at a dose of 30 mg kg −1 body weight in a small volume (0.2 ml) per injection. The mice were then subjected to I/R surgery. For I/R injury model, mice were subjected to 45 min ischaemia, then 3 h or 1 week reperfusion. We anaesthetized the animals, opened the chest and exposed the heart to identify the left anterior descending coronary artery. We passed a silk suture around the left anterior descending coronary artery at the inferior border of left auricle and occluded the artery by snaring with a vinyl tube through which the ligature had been passed. We occluded the coronary artery by pulling the snare tight and securing it with a hemostat. After 45 min of ischaemia, we released the ligature and reperfused the heart. Pink1-transgenic mice, miR-421-transgenic mice, E2F1 KO mice and WT mice were subjected to 45 min ischaemia, then 3 h or 1 week reperfusion. Sham-operated group experienced the same procedure except the snare was left untied. After 3 h of reperfusion, evans blue dye (1 ml of a 2.0% solution; Sigma-Aldrich) was injected into jugular vein into the heart for delineation of the ischaemic zone from the non-ischaemic zone. The heart was rapidly excised. The heart slices were incubated in 1.0% 2,3,5-triphenyltetrazolium chloride (Sigma-Aldrich) for 15 min at 37 °C for demarcation of the viable and non-viable myocardium within the risk zone. The staining was stopped by ice-cold sterile saline and the slices were fixed in 10% neutral buffered formaldehyde and individually weighed. Both sides of each slice were photographed. The areas of infarction and non-ischaemic left ventricle were assessed with computer-assisted planimetry (NIH Image 1.57) by an observer blinded to the sample identity. The ratio of infarction/left ventricle was calculated. Echocardiographic assessment Transthoracic echocardiographic analysis was performed on mice after 1 week of the sham or I/R surgery. We obtained echocardiographic parameters including systolic left ventricular internal diameters (LVIDs) and diastolic left ventricular internal diameters (LVIDd). We calculated fractional shortening of left ventricular diameter as [(LVIDd−LVIDs)/LVIDd] × 100. After in vivo evaluation of cardiac function, the mice were euthanized and the hearts were harvested, weighted and used for histological examination. Statistical analysis Data are expressed as the mean±s.e.m. of at least three independent experiments for each cellular experimental group and at least five independent experiments for each animal group. We evaluated the data with Student’s t -test. We used a one-way analysis of variance for multiple comparisons. A value of P <0.05 was considered significant. P.–F.L., J.Z. and K.W. designed the research. K.W., L.-Y.Z., J.-X.W., B.Z., T.A., B.L., N.L., T.S. and Y.W. performed the cellular experiments. K.W., Y.-J.Y., Y.G., J.-N.G. and Y.-H.D. conducted the animal experiments. P.-F.L. and K.W. wrote the manuscript. How to cite this article: Wang, K. et al . E2F1-dependent miR-421 regulates mitochondrial fragmentation and myocardial infarction by targeting Pink1. Nat. Commun . 6:7619 doi: 10.1038/ncomms8619 (2015).